Epigenetic plasticity ofCd8alocus during CD8+T-cell development and effector differentiation and reprogramming Modulation of CD8 coreceptor levels can profoundly affect T-cell sensitivity to antigen. Here we show that the heritable downregulation of CD8 during type 2 polarization of murine CD8 + effector T cells in vitro and in vivo is associated with CpG methylation of several regions of the Cd8a locus. These epigenetic modifications are maintained long-term in vivo following adoptive transfer. Even after extended type 2 polarization, however, some CD8 low effector cells respond to interferon-γ by re-expressing CD8 and a type 1 cytokine profile in association with partial Cd8a demethylation. Cd8a methylation signatures in naive, polarized and repolarized cells are distinct from those observed during the initiation, maintenance and silencing of CD8 expression by developing T cells in the thymus. This persistent capacity for epigenetic reprogramming of coreceptor levels on effector CD8 + T cells enables the heritable tuning of antigen sensitivity in parallel with changes in type 1/type 2 cytokine balance. The responsiveness of CD8 + T cells to peptide-class I MHC complexes (pMHCI) displayed on antigen-presenting cells can be strongly enhanced by interaction of the CD8αβ coreceptor with MHCI. By stabilizing TCR-pMHCI binding and augmenting TCR signalling [1] , [2] , [3] , [4] , [5] , CD8 can increase T-cell sensitivity to antigen by up to a million-fold, enabling responses to low-affinity and low-dose antigens [6] , [7] , [8] . Even small alterations in CD8 expression can therefore affect CD8 + T-cell responses profoundly. Expression of the CD8 coreceptor undergoes marked changes in thymocytes and peripheral CD8 + T cells according to developmental stage and activation state. During T-cell development, CD8 − CD4 − double-negative (DN) thymocytes first become CD8 + CD4 + double positive (DP) then undergo CD8 + or CD4 + T-cell lineage choice [9] . Various signals regulate CD8 levels on peripheral CD8 + T cells, allowing dynamic tuning of immune responsiveness [10] , [11] , [12] . TCR activation triggers transient CD8 downregulation without altering C d8a or C d8b mRNA levels [13] . As the CD8α subunit is essential for cell-surface expression of the CD8αβ heterodimer [14] , regulation of this subunit alone is sufficient to modulate CD8αβ levels. In the absence of TCR stimulation, the common γ-chain (γc) cytokines interleukin-2 (IL-2), IL-4, IL-7 and IL-15 increase CD8 levels on naive CD8 + T cells in vitro by increasing C d8a (but not C d8b ) transcription [12] . In contrast, IL-4 exposure during primary TCR-dependent activation in several different models causes progressive, sustained downregulation of C d8a mRNA and surface CD8, accompanied by a reduction in antigen sensitivity, induction of a type 2 cytokine profile and poor cytolytic function [15] , [16] , [17] , [18] ; interferon-γ (IFN-γ) antagonizes these effects [18] , [19] . With extended IL-4 exposure, essentially all activated CD8 + T cells acquire the type 2 CD8 low phenotype, which is then maintained over multiple cell divisions in the absence of IL-4 (ref. 17 ). The molecular mechanisms underpinning the stable inheritance of this phenotype and the potential for IFN-γ to reverse this heritable state have not previously been investigated. Methylation of DNA at CpG sites promotes gene silencing by establishing repressive chromatin states and restricting DNA accessibility to cellular machinery [20] . Changes in CpG methylation at specific genes facilitate heritable programming of lineage-specific gene expression profiles during differentiation. The murine Cd8a gene comprises five exons with five upstream enhancer regions (E8 I–V ) that regulate CD8 coreceptor expression in developing and mature CD8 + T cells [21] , [22] , [23] , [24] , [25] , [26] . An early study using restriction enzyme digestion showed that demethylation of seven CpG sites at the Cd8a locus occurs as thymocytes differentiate from DN to DP cells [27] . Later studies of E8 V , the distal promoter and gene body of Cd8a in DP-stage thymocytes lacking E8 I and E8 II found an association between demethylation of specific sites within E8 v and onset of CD8 expression [28] . Furthermore, mice lacking the maintenance DNA methyltransferase Dnmt1 showed impaired repression of CD8 expression on some TCRγδ + cells [29] . These findings suggest a role for CpG methylation in regulating CD8 expression during T-cell development. Whether it also contributes to heritable Cd8a gene silencing in peripheral CD8 low T cells is not known. We have now investigated how patterns of CpG methylation at various regions of the Cd8a locus change over the full course of normal T-cell development, primary activation and cytokine polarization in vitro and in vivo . We show that changes in CD8 expression in each of these circumstances are associated with distinct methylation patterns in and around the Cd8a gene. We further provide the first demonstration that epigenetic changes observed at Cd8a in differentiated effector CD8 + T cells are not fixed and, along with cytokine and granzyme expression profiles, can be reprogrammed. These results reveal unexpected epigenetic and functional plasticity in polarized effector CD8 + T cells that enables them to tune antigen sensitivity in parallel with repolarization of effector gene expression. Changes in DNA methylation at Cd8a during T-cell ontogeny To examine CpG methylation during the developmental programme of CD8 coreceptor expression in T cells, we extended earlier studies [27] , [28] , [29] to analyse methylation of 56 selected CpG sites across ~7.5 kb of the Cd8a locus, including 26 sites not previously examined, at key stages of thymic differentiation in normal mice. The sites were located within the E8 V enhancer, distal promoter, transcription start site (TSS) and two intragenic (IG) regions, IG1 and IG2 ( Fig. 1a ). Previously unstudied CpG sites at the TSS were selected because of its importance in transcription initiation. A CpG-rich intragenic region containing a cluster of eleven CpG dinucleotides within a stretch of 26 nucleotides (IG2) was identified and examined as intragenic DNA methylation has been correlated with gene expression [30] . 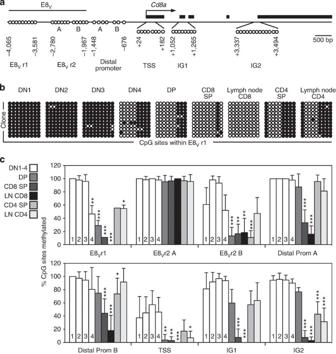Figure 1: Changes in DNA methylation atCd8acorrelate with CD8 expression during T-cell development. (a) Map of theCd8alocus, including the enhancer E8V(regions 1 (E8Vr1), 2A (E8Vr2A) and 2B (E8Vr2B)), distal promoter (regions A and B), transcription start site (TSS) and intragenic regions 1 (IG1) and 2 (IG2). Exons are represented by black rectangles and surveyed CpG sites by circles; the arrow marks the transcription start site. (b) CpG methylation of the 3′ distal portion of the CD8 enhancer E8Vin the indicated thymocyte and mature lymph node T-cell populations. Genomic DNA was bisulphite-modified, E8Vr1 was amplified by PCR, and products were cloned and sequenced. Open circles represent nonmethylated, and filled circles represent methylated CpG sites; rows represent individual clones; columns represent individual CpG sites within E8Vr1. (c) DNA methylation levels at E8Vr1 and seven other regions (indicated on thexaxis) in the same experiment asb(mean percentage±s.d. of CpG sites methylated in each region,n=at least 10 clones per population at each region). For each region, significant differences in % CpG methylation relative to DN1 cells were determined using a Kruskal–Wallis test followed by Dunn’spost test(*P<0.05, **P<0.01, ***P<0.001) (representative of two independent experiments). LN, lymph node. Figure 1: Changes in DNA methylation at Cd8a correlate with CD8 expression during T-cell development. ( a ) Map of the Cd8a locus, including the enhancer E8 V (regions 1 (E8 V r1), 2A (E8 V r2A) and 2B (E8 V r2B)), distal promoter (regions A and B), transcription start site (TSS) and intragenic regions 1 (IG1) and 2 (IG2). Exons are represented by black rectangles and surveyed CpG sites by circles; the arrow marks the transcription start site. ( b ) CpG methylation of the 3′ distal portion of the CD8 enhancer E8 V in the indicated thymocyte and mature lymph node T-cell populations. Genomic DNA was bisulphite-modified, E8 V r1 was amplified by PCR, and products were cloned and sequenced. Open circles represent nonmethylated, and filled circles represent methylated CpG sites; rows represent individual clones; columns represent individual CpG sites within E8 V r1. ( c ) DNA methylation levels at E8 V r1 and seven other regions (indicated on the x axis) in the same experiment as b (mean percentage±s.d. of CpG sites methylated in each region, n =at least 10 clones per population at each region). For each region, significant differences in % CpG methylation relative to DN1 cells were determined using a Kruskal–Wallis test followed by Dunn’s post test (* P <0.05, ** P <0.01, *** P <0.001) (representative of two independent experiments). LN, lymph node. Full size image Genomic DNA from purified populations of DN stages 1–4 (ref. 9 ), DP, CD4 single positive (SP) and CD8 SP thymocytes, and naive CD8 + and CD4 + lymph node T cells, was bisulphite treated, and the Cd8a regions identified above were PCR amplified, cloned and sequenced to determine CpG methylation status ( Fig. 1b,c and Supplementary Fig. 1 ). DN1, 2 and 3 thymocytes exhibited methylation of most (typically >90%) CpG cytosines within E8 V , the distal promoter, IG1 and IG2, and heterogeneous methylation at the TSS (range 0–100%). With transition through DN4 to the DP stage when CD8 is first expressed, there was a progressive reduction in methylation within two regions of E8 V (spanning −4,065 to −3,657 bp [E8 V r1] and −2,266 to −2,056 bp [E8 V r2B]) and almost complete loss (<5% remaining) at the TSS. The demethylation of particular CpG sites within E8 V in DP thymocytes confirms previous findings [28] . In addition, the data show that demethylation begins at DN4, before initiation of CD8 expression. With differentiation of DP thymocytes into CD8 SP cells, methylation was further reduced at E8 V r1 and the distal promoter, and mostly lost (<20% remaining) at intragenic regions. Thus, CD8 SP thymocytes displayed little methylation (<10% mean) within the Cd8a gene. This pattern was maintained in peripheral CD8 + T cells, with further reductions in methylation at some regions. CD4 SP thymocytes that had silenced CD8 expression maintained high methylation levels at the distal promoter (>70% mean) and intermediate levels at IG1 (57.2±21.0%), similar to DP thymocytes (60.0±20.7%). CD4 SP thymocytes also remethylated some cytosines within E8 V and at the TSS. Peripheral CD4 + T cells largely maintained this pattern. E8 V r2A remained highly methylated (>95% mean) at all stages. Overall, the data demonstrate that significant changes in DNA methylation at multiple regions of the Cd8a locus correlate with the initiation, maintenance and silencing of Cd8a expression in developing T cells. Notably, each developmental stage from DN3 onwards was marked by a unique CpG methylation profile. These patterns were highly reproducible and, with previous studies [28] , suggest a role for CpG methylation in regulating CD8 expression. Increased DNA methylation at Cd8a in type 2 CD8 low cells Activation of naive CD8 + T cells in the presence of IL-4 leads to marked downregulation of Cd8a mRNA and cell surface CD8 coreceptor expression [16] , [18] , which then remains low or undetectable through multiple cell divisions in vitro and in vivo in the absence of IL-4 (refs 17 , 31 ). The stable and heritable nature of this loss of CD8 expression suggests that IL-4 might induce epigenetic changes to the Cd8a locus. To test whether CpG methylation profiles at Cd8a changed following polarization, naive lymph node CD8 + T cells were activated with immobilized antibodies to CD3ε, CD8α and CD11a (anti-receptor Ab) in the presence of IL-2 alone (neutral conditions) or with IL-2, IL-4 and neutralizing anti-IFN-γ Ab (type 2 polarizing conditions). Almost every naive CD8 + T cell is activated to proliferate and undergo effector differentiation in this system [16] , [32] . As previously reported [17] , [18] , cells activated in type 2 conditions progressively downregulated surface CD8α expression between days 4 and 10, while most cells activated in neutral conditions retained high CD8 levels ( Fig. 2a ). This loss of CD8 in cultures with IL-4 was STAT6 dependent as STAT6 −/− CD8 + T cells activated in type 2 conditions did not downregulate CD8 below the levels seen in neutral cultures. CD8 low cells in type 2 cultures expressed similar CD62L levels, somewhat reduced CD44 and delayed upregulation of PD-1 compared with CD8 high cells from neutral cultures ( Supplementary Fig. 2a ). Unlike IL-4, IL-13 did not cause downregulation of CD8 or upregulation of the type 2 transcription factor GATA-3 during primary CD8 + T-cell activation ( Supplementary Fig. 2b,c ). 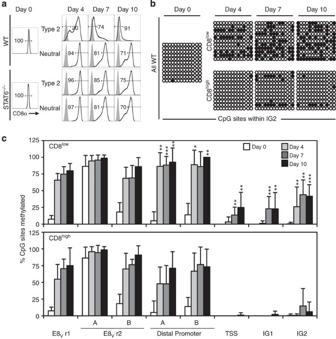Figure 2: IL-4-induced loss of CD8 expression during primary CD8+T-cell activation is STAT6 dependent and associated with increased DNA methylation atCd8a. (a) Surface CD8α levels before and after activation of naive lymph node CD8+T cells from wild-type or STAT-6−/−mice with immobilized Ab to CD3ε, CD8 and CD11a, in the presence of IL-2, IL-4 and anti-IFN-γ Ab (type 2 conditions) or IL-2 alone (neutral conditions) (grey: isotype control). (b) Methylation atCd8aIG2 in wild type naive CD8+T cells (day 0) and type 2 CD8lowcells and neutral CD8highcells after activation for 4, 7 or 10 days as ina. (c) Methylation levels across theCd8alocus in type 2 CD8lowcells (upper panel) and neutral CD8highcells (lower panel) (mean percentage±s.d. of CpG sites methylated in each region;n=at least 10 clones per population at each region; *P<0.05, **P<0.01, ***P<0.001 by Mann–Whitney test comparing CD8lowand CD8highcells for each region at each time point). The day 0 starting population is included in both panels. Data are representative of at least two independent experiments. Figure 2: IL-4-induced loss of CD8 expression during primary CD8 + T-cell activation is STAT6 dependent and associated with increased DNA methylation at Cd8a. ( a ) Surface CD8α levels before and after activation of naive lymph node CD8 + T cells from wild-type or STAT-6 −/− mice with immobilized Ab to CD3ε, CD8 and CD11a, in the presence of IL-2, IL-4 and anti-IFN-γ Ab (type 2 conditions) or IL-2 alone (neutral conditions) (grey: isotype control). ( b ) Methylation at Cd8a IG2 in wild type naive CD8 + T cells (day 0) and type 2 CD8 low cells and neutral CD8 high cells after activation for 4, 7 or 10 days as in a . ( c ) Methylation levels across the Cd8a locus in type 2 CD8 low cells (upper panel) and neutral CD8 high cells (lower panel) (mean percentage±s.d. of CpG sites methylated in each region; n =at least 10 clones per population at each region; * P <0.05, ** P <0.01, *** P <0.001 by Mann–Whitney test comparing CD8 low and CD8 high cells for each region at each time point). The day 0 starting population is included in both panels. Data are representative of at least two independent experiments. Full size image CpG methylation at Cd8a was analysed in CD8 low cells from type 2 cultures and CD8 high cells from neutral cultures at days 4, 7 and 10 following activation ( Fig. 2b,c and Supplementary Fig. 3 ). CD8 low and CD8 high cells displayed increased methylation at E8 V and the distal promoter at all time points compared with naive CD8 + T cells. However, CD8 low cells displayed significantly higher levels of methylation at the promoter than CD8 high cells at most time points. CpG methylation also increased at the TSS and intragenic regions of CD8 low cells over time; these regions remained largely demethylated in CD8 high cells. There was substantial clonal heterogeneity in the levels and patterns of CpG methylation at the TSS and intragenic regions of CD8 low cells ( Fig. 2b , Supplementary Fig. 3 ). Nevertheless, after 10 days in type 2 culture, most (75–100%) CD8 low cells displayed some methylation at these regions, whereas few (10–40%) CD8 high cells from neutral cultures showed any methylation. Interestingly, methylation patterns were similar in CD8 low cells, CD4 SP thymocytes and peripheral CD4 + T cells (comparing Figs 1c and 2c ). The results show that CD8 + T-cell activation in neutral or type 2 conditions induces distinct changes in CpG methylation at Cd8a . The strong correlation between IL-4-induced CD8 downregulation in primary activated CD8 + T cells and increased CpG methylation at the Cd8a distal promoter, TSS and intragenic regions is consistent with a role for DNA methylation in Cd8a gene silencing in these cells. Increased Cd8a methylation in CD8 low cells induced in vivo We have previously shown CD8 downregulation and type 2 polarization of IFN-γ-deficient ovalbumin (OVA)-specific TCR transgenic OT-I cells activated in vivo in response to a tumour expressing OVA and IL-4 (refs 18 , 19 ). To determine whether CD8 low cells generated in similar conditions in vivo also displayed altered DNA methylation at the Cd8a locus, OT-I CD8 + T cells were adoptively transferred into anti-IFN-γ Ab-treated recipient mice with an IL-4-expressing OVA + tumour (type 2 conditions) or into untreated recipients with control OVA + tumour (neutral conditions) ( Fig. 3 ). At day 9, CD8 was partially downregulated on OT-I cells activated in type 2 conditions, and CpG methylation at the four most informative regions of Cd8a was significantly higher in purified CD8 low cells from these mice than in CD8 high cells activated in vivo in the absence of IL-4 and anti-IFN-γ Ab. The patterns of methylation observed in vivo were similar to those shown in CD8 low and CD8 high cells activated in vitro in type 2 and neutral conditions, respectively (compare Fig. 3 with Fig. 2 and Supplementary Fig. 3 ). The data suggest that IL-4-dependent downregulation of CD8 is associated with increased methylation of the Cd8a locus in vivo as well as in vitro . 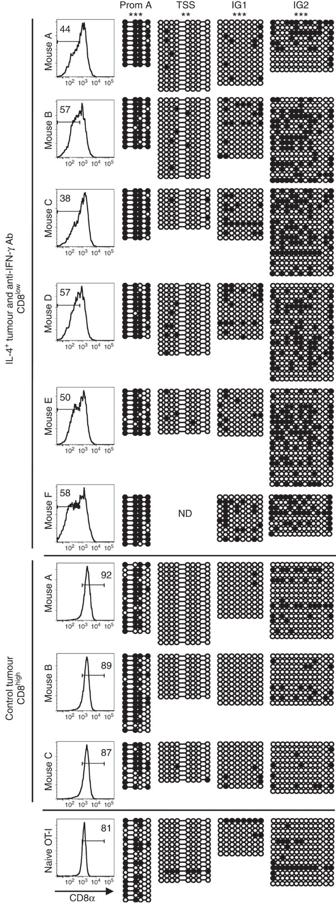Figure 3: CD8lowT cells generatedin vivodisplay increased methylation ofCd8a. CD8+T cells from OT-I mice were coinjected with OVA-expressing EG7-IL-4+or EG7-IL-4−(control) tumour cells into RAG-2−/−γc−/−mice. EG7-IL-4+tumour recipients also received anti-IFN-γ mAb on days 0, 4 and 6. On day 9, Vα2+CD4−CD8lowand CD8highsplenocytes were purified from mice that received EG7-IL-4+and control tumour, respectively, and DNA was extracted for CpG methylation analysis. Rows represent individual clones; circles represent unmethylated (open) and methylated (filled) CpG sites. **P<0.01, ***P<0.001 by χ2-test comparing percentages of CpG sites methylated at each region in CD8lowcells (n=6 mice) and CD8highcells (n=3 mice). ND, no data available. Figure 3: CD8 low T cells generated in vivo display increased methylation of Cd8a . CD8 + T cells from OT-I mice were coinjected with OVA-expressing EG7-IL-4 + or EG7-IL-4 − (control) tumour cells into RAG-2 −/− γc −/− mice. EG7-IL-4 + tumour recipients also received anti-IFN-γ mAb on days 0, 4 and 6. On day 9, Vα2 + CD4 − CD8 low and CD8 high splenocytes were purified from mice that received EG7-IL-4 + and control tumour, respectively, and DNA was extracted for CpG methylation analysis. Rows represent individual clones; circles represent unmethylated (open) and methylated (filled) CpG sites. ** P <0.01, *** P <0.001 by χ 2 -test comparing percentages of CpG sites methylated at each region in CD8 low cells ( n =6 mice) and CD8 high cells ( n =3 mice). ND, no data available. Full size image Maintenance of methylation at Cd8a in CD8 low cells in vivo To examine the stability of the changes in CpG methylation observed in CD8 low cells, naive CD45.1 + CD8 + T cells were activated in neutral or type 2 conditions for 7 days, then recultured in IL-2 alone for 2 days. CD8 low cells from type 2 cultures and CD8 high cells from neutral cultures were then adoptively transferred into CD45.2 + congenic mice. After 62 days in vivo , substantially greater numbers of CD45.1 + donor cells were recovered from mice that received CD8 low cells compared with CD8 high cells ( Fig. 4a ). This result was obtained whether or not cells were recultured in IL-2 before transfer to allow loss of surface-bound anti-CD8α Ab ( Supplementary Table 1 ), suggesting that the lower recovery of CD8 high cells was not due to Ab-mediated deletion in vivo ; instead, CD8 low -cell survival may have been enhanced by IL-4 exposure during activation [33] . 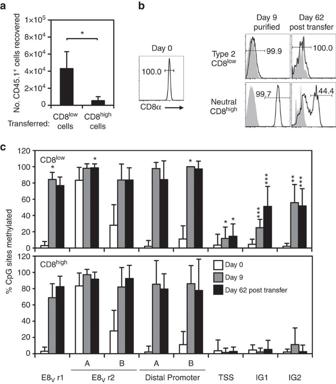Figure 4: CD8lowcells are stable long-termin vivoand maintain patterns of increased DNA methylation atCd8a. (a) Recovery of donor CD45.1+cells 62 days after adoptive transfer of CD8lowcells from type 2 cultures or CD8highcells from neutral cultures into CD45.2+mice (mean±s.d. per mouse) (*P=0.0328, comparing CD8lowand CD8highrecipient groups by two-tailedt-test). (b) Surface CD8α expression by naive CD8+T cells (day 0) andin vitroactivated T cells before (day 9) and 62 days after adoptive transfer (grey: isotype control). (c) DNA methylation levels atCd8ain naive CD8+T cells and CD8lowand CD8highcells before and after adoptive transfer (mean percentage±s.d. of CpG sites methylated in each region;n=at least 10 clones per population at each region *P<0.05, **P<0.01, ***P<0.001 by Mann–Whitney test comparing CD8lowand CD8highcells for each region) (representative of two independent experiments). Figure 4: CD8 low cells are stable long-term in vivo and maintain patterns of increased DNA methylation at Cd8a. ( a ) Recovery of donor CD45.1 + cells 62 days after adoptive transfer of CD8 low cells from type 2 cultures or CD8 high cells from neutral cultures into CD45.2 + mice (mean±s.d. per mouse) (* P =0.0328, comparing CD8 low and CD8 high recipient groups by two-tailed t -test). ( b ) Surface CD8α expression by naive CD8 + T cells (day 0) and in vitro activated T cells before (day 9) and 62 days after adoptive transfer (grey: isotype control). ( c ) DNA methylation levels at Cd8a in naive CD8 + T cells and CD8 low and CD8 high cells before and after adoptive transfer (mean percentage±s.d. of CpG sites methylated in each region; n =at least 10 clones per population at each region * P <0.05, ** P <0.01, *** P <0.001 by Mann–Whitney test comparing CD8 low and CD8 high cells for each region) (representative of two independent experiments). Full size image CD8 low cells recovered 62 days after transfer maintained low CD8 levels similar to their profiles before transfer, illustrating the long-term stability of this phenotype [17] , [31] , whereas CD8 high cells displayed variable CD8 levels ( Fig. 4b ). CpG methylation analysis of naive and 9-day in vitro activated CD8 low and CD8 high cells ( Fig. 4c and Supplementary Fig. 4 ) gave similar results to those above ( Figs 2c and 3 ), except that methylation of the distal promoter set A was comparable in CD8 low and CD8 high cells. Most remarkably, the methylation profiles of 9-day CD8 low and CD8 high cells were maintained in cells rested in vivo for 62 days then sorted for low or high CD8 expression; the only exception was a significant increase in IG1 methylation in CD8 low cells after adoptive transfer ( P =0.0089). These data indicate that in vitro activation of naive CD8 + T cells under neutral or type 2 conditions induces distinct and stable changes in CpG methylation at the Cd8a locus that are maintained in vivo in the absence of high-affinity TCR stimulation. Notably, the long-term stability of the CD8 low phenotype correlated with maintenance of increased CpG methylation at the TSS and intragenic regions. This suggests that IL-4 exposure during primary activation induces stable commitment to a CD8 low phenotype through epigenetic silencing of the Cd8a locus. Plasticity of CD8 low phenotype in polarized effector cells IFN-γ counteracts IL-4-induced CD8 downregulation during primary CD8 + T-cell effector differentiation in vivo and in vitro [18] . To test whether IFN-γ could also act later to reverse CD8 downregulation in type 2-polarized CD8 low cells, in vitro generated CD8 low cells were restimulated with anti-receptor Ab and IL-2 with or without IFN-γ, IL-4 and/or anti-cytokine Ab for 8 days ( Fig. 5a ). CD8 low cells restimulated in type 2 (IL-4 and anti-IFN-γ Ab) or neutral conditions (none) remained CD8 low as previously reported [17] . In neutralizing concentrations of anti-IL-4 Ab, a small proportion of cells (6.3%) re-expressed CD8, suggesting that endogenous IL-4 maintained the CD8 low phenotype of some cells under neutral conditions. IFN-γ induced CD8 re-expression on 34% of cells, but CD8 re-expression was highest (41%) when both IFN-γ and anti-IL-4 Ab were present. CD8 was re-expressed as CD8αβ heterodimers ( Supplementary Fig. 5a ). Thus, IFN-γ and IL-4 reciprocally regulate CD8 expression not only during primary CD8 + T-cell activation [18] , [19] but also during restimulation of type 2-polarized CD8 low cells. 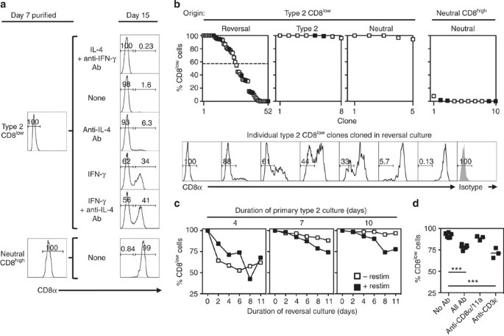Figure 5: IFN-γ induces CD8 re-expression on some CD8lowcells. (a) Surface CD8 expression by 7-day type 2 CD8lowcells and neutral CD8highcells before and after purification and restimulation with anti-receptor Ab and IL-2 for 8 days in the indicated conditions. (b) CD8 expression by clones grown from single twice-purified 7-day type 2 CD8lowcells and neutral CD8highcells cultured with anti-receptor Ab and IL-2 in reversal (IFN-γ and anti-IL-4 Ab), type 2 or neutral conditions for 13 days. Cells expanded 911-fold during primary activation (≥9–10 cell divisions). Cloning efficiencies were CD8low→reversal, 13.1%; CD8low→type 2, 6.6%; CD8low→neutral, 14.3%; CD8high→neutral, 15.8%. Upper panels show clones estimated to contain ≥100 cells from two independent experiments (filled and empty symbols) ranked by % CD8lowcells (dashed line: median % CD8low). Lower panels show representative CD8lowclones cultured in reversal conditions (isotype control staining of pooled clones in grey). (c) Percent CD8lowcells among twice-purified CD8lowcells from primary type 2 cultures after re-culture in reversal conditions with or without anti-receptor Ab (n=3, except day 4 primary cells re-cultured for 2 days with (n=2) or without (n=1) restimulation) (representative of three independent experiments). (d) Percent CD8lowcells among twice-purified CD8lowcells from 7-day type 2 cultures after re-culture for 8 days in reversal conditions with the indicated immobilized Ab (***P<0.001, one-way ANOVA with Bonferroni’s post test for multiple comparisons) (representative of three independent experiments). Figure 5: IFN-γ induces CD8 re-expression on some CD8 low cells. ( a ) Surface CD8 expression by 7-day type 2 CD8 low cells and neutral CD8 high cells before and after purification and restimulation with anti-receptor Ab and IL-2 for 8 days in the indicated conditions. ( b ) CD8 expression by clones grown from single twice-purified 7-day type 2 CD8 low cells and neutral CD8 high cells cultured with anti-receptor Ab and IL-2 in reversal (IFN-γ and anti-IL-4 Ab), type 2 or neutral conditions for 13 days. Cells expanded 911-fold during primary activation (≥9–10 cell divisions). Cloning efficiencies were CD8 low →reversal, 13.1%; CD8 low →type 2, 6.6%; CD8 low →neutral, 14.3%; CD8 high →neutral, 15.8%. Upper panels show clones estimated to contain ≥100 cells from two independent experiments (filled and empty symbols) ranked by % CD8 low cells (dashed line: median % CD8 low ). Lower panels show representative CD8 low clones cultured in reversal conditions (isotype control staining of pooled clones in grey). ( c ) Percent CD8 low cells among twice-purified CD8 low cells from primary type 2 cultures after re-culture in reversal conditions with or without anti-receptor Ab ( n =3, except day 4 primary cells re-cultured for 2 days with ( n =2) or without ( n =1) restimulation) (representative of three independent experiments). ( d ) Percent CD8 low cells among twice-purified CD8 low cells from 7-day type 2 cultures after re-culture for 8 days in reversal conditions with the indicated immobilized Ab (*** P <0.001, one-way ANOVA with Bonferroni’s post test for multiple comparisons) (representative of three independent experiments). Full size image It was possible that the re-emergence of CD8 + cells in secondary cultures of CD8 low cells was due to outgrowth of rare contaminating CD8 high cells. To determine directly whether CD8 low cells could re-express CD8, individual twice-purified CD8 low cells from type 2 cultures and CD8 high cells from neutral cultures were restimulated with anti-receptor Ab and IL-2 in reversal (IFN-γ and anti-IL-4 Ab), type 2 or neutral conditions and clones of ≥100 cells were examined 13 days later. Of 52 CD8 low clones in reversal conditions, 43 contained CD8-expressing daughter cells ( Fig. 5b ). Although the proportion of CD8 + cells varied greatly between clones (range 0–100%, median CD8 low 57.3%), there was no apparent correlation with clone size ( Supplementary Fig. 5b ), suggesting that CD8 + cell frequency was not linked to division number. Control CD8 low clones cultured in type 2 or neutral conditions largely maintained a CD8 low phenotype, and CD8 high clones from neutral conditions were mostly CD8 high . The data confirm the potential of some CD8 low cells to re-express CD8 in response to IFN-γ. We next examined the requirements for optimal CD8 re-expression. The frequency of CD8-expressing cells was highest when CD8 low cells were transferred from primary type 2 cultures to reversal conditions after only 4 days compared with day 7 or 10 ( Fig. 5c ), suggesting that longer exposure to type 2 stimuli stabilizes commitment to a CD8 low phenotype. At the later time points, CD8 re-expression was enhanced by anti-receptor Ab stimulation. This effect depended on TCR ligation: CD8 re-expression was higher in reversal conditions with all three anti-receptor Ab or with anti-CD3ε Ab alone than with anti-CD8α/CD11a or no Ab ( Fig. 4d ). Association of CD8 re-expression and effector reprogramming As well as reciprocally modulating CD8 expression, IL-4 promotes and IFN-γ counteracts the induction of type 2 cytokine synthesis and loss of cytolytic function in CD8 + T cells [19] . We therefore investigated whether reversal of the CD8 low phenotype by IFN-γ was accompanied by modulation of type 2 effector function. After primary activation in type 2 conditions, most cells were CD8 low (86%) and produced IL-4 (50%) but not IFN-γ (0.2% positive) or granzyme B (GzmB; 26% positive), whereas most cells in neutral cultures maintained CD8 expression and produced IFN-γ (76%) and GzmB (55%) but not IL-4 (0.3%) ( Fig. 6a ), consistent with previous reports [16] , [19] . Restimulation of type 2-polarized CD8 low cells under reversal conditions for 10 days resulted in CD8 re-expression on ~22% of cells ( Fig. 6b ). Compared with CD8 low cells from the same cultures, this CD8 + population displayed reduced IL-4 and significant upregulation of IFN-γ and GzmB to proportions seen in neutral effector cells maintained in neutral culture ( Fig. 6b,c ). Thus, CD8 re-expression was associated with a loss of type 2 polarization and a shift towards a type 1 effector phenotype. In contrast, CD8 high cells continued in neutral cultures and CD8 low cells continued in type 2 conditions maintained type 1 and type 2 effector phenotypes, respectively. 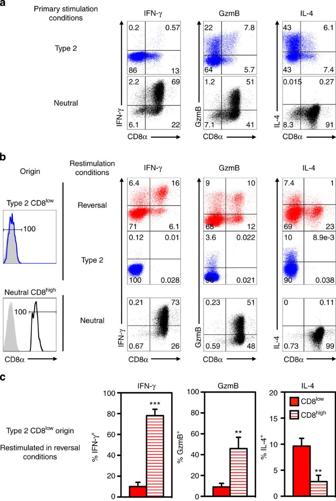Figure 6: Reversal of CD8 phenotype is accompanied by a switch to a type 1 effector phenotype. (a) Primary culture: intracellular IFN-γ, GzmB and IL-4 expression by CD8+T cells after activation in type 2 or neutral conditions for 7 days, culture in IL-2 for 2 days, then restimulation with PMA, ionomycin and monensin for 4 h. (b) Secondary culture: intracellular IFN-γ, GzmB and IL-4 expression by twice-purified CD8lowcells from 7-day type 2 cultures (upper left panel, isotype control in grey) re-cultured for 10 days in reversal (IL-2, IFN-γ and anti-IL-4 Ab) or type 2 conditions, IL-2 for 3 days, then PMA, ionomycin and monensin for 4 h. Purified CD8highcells from 7-day neutral cultures (lower left panel) were re-stimulated in neutral conditions. (c) Frequencies of IFN-γ, GzmB and IL-4 producing CD8lowand CD8highcells in reversal cultures (mean±s.d.,n=three independent reversal cultures; **P<0.01, ***P<0.001 by two-tailedt-test) (representative of two independent experiments). Figure 6: Reversal of CD8 phenotype is accompanied by a switch to a type 1 effector phenotype. ( a ) Primary culture: intracellular IFN-γ, GzmB and IL-4 expression by CD8 + T cells after activation in type 2 or neutral conditions for 7 days, culture in IL-2 for 2 days, then restimulation with PMA, ionomycin and monensin for 4 h. ( b ) Secondary culture: intracellular IFN-γ, GzmB and IL-4 expression by twice-purified CD8 low cells from 7-day type 2 cultures (upper left panel, isotype control in grey) re-cultured for 10 days in reversal (IL-2, IFN-γ and anti-IL-4 Ab) or type 2 conditions, IL-2 for 3 days, then PMA, ionomycin and monensin for 4 h. Purified CD8 high cells from 7-day neutral cultures (lower left panel) were re-stimulated in neutral conditions. ( c ) Frequencies of IFN-γ, GzmB and IL-4 producing CD8 low and CD8 high cells in reversal cultures (mean±s.d., n =three independent reversal cultures; ** P <0.01, *** P <0.001 by two-tailed t -test) (representative of two independent experiments). Full size image The data show that a combination of TCR triggering, IFN-γ exposure and lack of IL-4 can induce CD8 re-expression and re-polarization towards type 1 effector function in some type 2-polarized CD8 low cells, suggesting that CD8 expression is one of a suite of functions that can be reprogrammed after primary effector differentiation. Loss of DNA methylation at Cd8a in re-polarized CD8 + T cells The cytosine methylation inhibitor 5-azacytidine was used to investigate the role of CpG methylation in generating and maintaining the CD8 low state. The presence of 5-azacytidine during primary CD8 + T-cell activation in type 2 conditions had no effect on CD8 expression ( Supplementary Fig. 6 ). By contrast, 5-azacytidine addition to reversal cultures substantially increased the proportion of CD8-expressing cells ( Fig. 7a ). This effect was reproducible in multiple experiments, but with variable dose dependence. A similar but more modest effect was observed in neutral cultures, suggesting that loss of CpG methylation can promote CD8 re-expression in some CD8 low cells in the absence of exogenous IFN-γ. 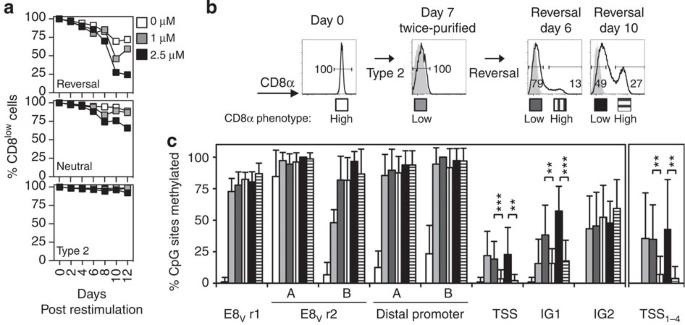Figure 7: Loss of DNA methylation atCd8acorrelates with the re-acquisition of CD8 expression. (a) Percent CD8lowcells in secondary cultures of 7-day type 2 CD8lowcells in the absence or presence of 1 mM or 2.5 mM 5-azacytidine (representative of three independent experiments). (b) CD8 expression by twice-purified CD8lowcells from 7-day type 2 cultures following restimulation in reversal conditions (IL-2, IFN-γ and anti-IL-4 Ab) with anti-receptor Ab for 6 or 10 days (isotype control in grey). (c) Methylation analysis of genomic DNA from the purified CD8lowand CD8highpopulations shown inb. The mean percentage (±s.d.) of methylated CpG sites within a region is shown; right hand panel shows data for the first four CpG sites at the TSS; comparison of methylation levels between cells that remained CD8lowin reversal culture and those that re-expressed CD8 in the same conditions (n=at least 10 clones per population at each region; **P<0.01, ***P<0.001 by Mann–Whitney test). Data are representative of two independent experiments. Figure 7: Loss of DNA methylation at Cd8a correlates with the re-acquisition of CD8 expression. ( a ) Percent CD8 low cells in secondary cultures of 7-day type 2 CD8 low cells in the absence or presence of 1 mM or 2.5 mM 5-azacytidine (representative of three independent experiments). ( b ) CD8 expression by twice-purified CD8 low cells from 7-day type 2 cultures following restimulation in reversal conditions (IL-2, IFN-γ and anti-IL-4 Ab) with anti-receptor Ab for 6 or 10 days (isotype control in grey). ( c ) Methylation analysis of genomic DNA from the purified CD8 low and CD8 high populations shown in b . The mean percentage (±s.d.) of methylated CpG sites within a region is shown; right hand panel shows data for the first four CpG sites at the TSS; comparison of methylation levels between cells that remained CD8 low in reversal culture and those that re-expressed CD8 in the same conditions ( n =at least 10 clones per population at each region; ** P <0.01, *** P <0.001 by Mann–Whitney test). Data are representative of two independent experiments. Full size image To analyse the effect of 5-azacytidine on proliferation in reversal cultures, CD8 low cells from primary type 2 cultures were stained with a division tracking dye before reversal culture with or without 5-azacytidine for 4 days ( Supplementary Fig. 7 ). While the effect of 5-azacytidine on CD8 expression was modest at day 4 (consistent with the data in Fig. 7a ), analysis at this early time point enabled the extent of cell division to be compared between cultures before complete dilution of the dye. On average 5-azacytidine reduced the apparent rate of proliferation (or increased death of the most divided cells) in reversal culture. As the full impact of 5-azacytidine requires at least two cell divisions [34] , this reduction in proliferation dampens its effects on reversal. The data show, however, that CD8 high cells had undergone more divisions on average than CD8 low cells in cultures with 5-azacytidine, consistent with CD8 re-expression being division dependent. Moreover, cells which had undergone two or more divisions in reversal cultures expressed higher CD8 levels in the presence of 5-azacytidine than in its absence, despite the fact that they had undergone fewer divisions beyond the second cycle. In summary, despite the limitations associated with the use of 5-azacytidine, the data suggest that DNA methylation is not responsible for the initial downregulation of CD8 but instead contributes to the maintenance of Cd8a gene silencing in established CD8 low cells. To determine whether re-expression of CD8 correlated with changes in DNA methylation at Cd8a , 7-day type 2-polarized CD8 low cells were cultured in reversal conditions with anti-receptor Ab for 6 or 10 days before analysis ( Fig. 7b ). Cells that maintained a CD8 low phenotype in reversal conditions displayed methylation profiles similar to those of the primary CD8 low population ( Fig. 7c and Supplementary Fig. 8a ). Most (>75% mean) CpG sites within E8 V and the distal promoter of these cells were methylated, and some CpG sites within the TSS, IG1 and IG2 were variably methylated. Interestingly, CD8 low cells from reversal cultures displayed higher levels of methylation at IG1 (38.2±23.7%, reversal day 6; 57.3±19.5%, reversal day 10) than the primary CD8 low population (15.6±19.3% day 7), increasing from day 6 to 10 in reversal conditions. Levels of methylation at IG1 of CD8 low cells from day 10 reversal cultures were similar to those in long-term CD8 low cells (comparing CD8 low reversal day 10 in Fig. 6c with CD8 low day 62 in Fig. 4c ). The data suggest that some CD8 low cells remain committed to a CD8 low phenotype, even in reversal conditions. No differences were detected in CpG methylation at E8 V , the distal promoter and IG2 of CD8-expressing and non-expressing cells from reversal cultures ( Fig. 7c and Supplementary Fig. 8 ). However, cells that regained CD8 expression displayed significantly less methylation at the TSS than CD8 low cells from reversal cultures and CD8 low cells from type 2 cultures. This difference was more pronounced when only the first four CpG sites at the TSS were considered (TSS 1–4 ) ( Fig. 7c ), demonstrating a strong correlation between demethylation of these sites and CD8 re-expression. This pattern of TSS demethylation was also observed in naive CD8 + T cells and neutral CD8 high cells ( Supplementary Fig. 8b ). CD8-re-expressing cells from reversal cultures also displayed less methylation at IG1 compared with CD8 low cells from reversal cultures ( Fig. 7c ), although this difference was only seen at day 6 in a repeat experiment and was less striking ( Supplementary Fig. 8b ). Notably, the methylation profiles of CD8-re-expressing cells differed from naive CD8 + T cells and CD8 high cells from neutral cultures, displaying higher mean levels of methylation at the distal promoter and intragenic regions at most time points ( Supplementary Fig. 8b ). Thus, unique methylation signatures were observed at the Cd8a locus at each stage of T-cell development in the thymus from the DN3 stage onwards, and in peripheral CD8 + T cells following primary activation, heritable CD8 silencing in type 2-polarized cells and subsequent type 1 re-polarization and CD8 re-expression ( Fig. 8 ). 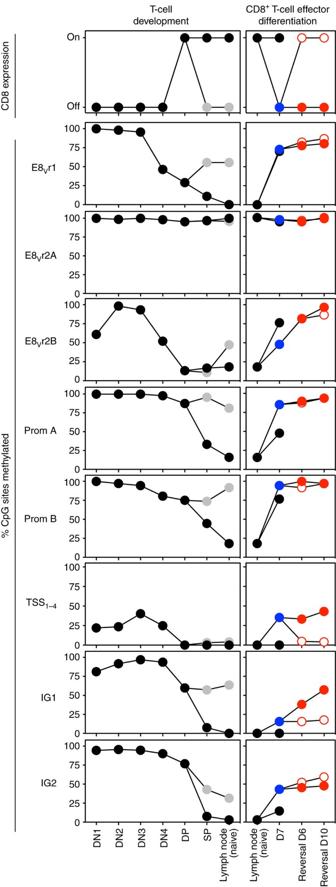Figure 8: Distinct DNA methylation signatures atCd8aare associated with different stages of T-cell differentiation. Surface CD8 phenotypes (uppermost panels) and mean percentage CpG sites methylated at the indicated regions of theCd8alocus during T-cell development (left panels: black symbol, CD8 lineage; grey, CD4 lineage) and CD8+T-cell effector differentiation and reprogramming (right panels: black, naive CD8+T cells and 7-day neutral CD8highcells; blue, 7-day type 2 CD8loweffector cells; red, type 2 CD8lowcells that remained CD8lowin secondary reversal culture; unfilled red, type 2 CD8lowcells that re-expressed CD8 in reversal culture). TSS1–4represents the first four CpG sites at theCd8aTSS. Figure 8: Distinct DNA methylation signatures at Cd8a are associated with different stages of T-cell differentiation. Surface CD8 phenotypes (uppermost panels) and mean percentage CpG sites methylated at the indicated regions of the Cd8a locus during T-cell development (left panels: black symbol, CD8 lineage; grey, CD4 lineage) and CD8 + T-cell effector differentiation and reprogramming (right panels: black, naive CD8 + T cells and 7-day neutral CD8 high cells; blue, 7-day type 2 CD8 low effector cells; red, type 2 CD8 low cells that remained CD8 low in secondary reversal culture; unfilled red, type 2 CD8 low cells that re-expressed CD8 in reversal culture). TSS 1–4 represents the first four CpG sites at the Cd8a TSS. Full size image Here we show that cytokine modulation of CD8 coreceptor levels on activated CD8 + T cells is associated with epigenetic modification of the Cd8a locus in vitro and in vivo , providing a mechanism to establish and maintain the set point for antigen sensitivity through many cell divisions. Some CD8 + effector cells can nevertheless be epigenetically and functionally reprogrammed, in contrast to the widely held view that they are committed to a type 1 cytotoxic phenotype. The initiation, maintenance, silencing and re-induction of CD8 coreceptor expression at different stages of thymic and peripheral T-cell differentiation correlated with distinct patterns of CpG methylation in and around the Cd8a locus. The data strongly suggest that DNA methylation is involved in regulating Cd8a gene expression in thymic and peripheral T cells. Changes in DNA methylation occurred gradually both before and after changes in CD8 expression but, once established, were maintained over long periods in vivo . Thus, while it might play a role in initiating activation of the Cd8a gene, it seems likely that DNA methylation primarily acts later to stabilize gene expression as part of a multi-step process in which binding of specific factors to the locus precedes the coordinate modification of chromatin structure, histone proteins and DNA methylation [20] . Of these steps, DNA methylation provides the most stable long-term gene repression [35] , [36] . Numerous transcription factors have been implicated in CD8 transcriptional control [12] , [28] , [37] , [38] , [39] and might be candidates to initiate this process. We show that the IL-4-induced downregulation of CD8 in primary activated CD8 + T cells depends on one of these factors, STAT6. The Cd8a locus contains multiple STAT6- and GATA3-binding sites within and between the CpG-rich regions analysed in this study (K.L.H. and E.B.D., unpublished observations). STAT6 activated in response to IL-4 might therefore act directly, or via induction of GATA3 (ref. 40 ), to initiate transcriptional repression of the Cd8a locus, with subsequent methylation of CpG sites across the locus helping to stabilize commitment to the CD8 low phenotype. Such a mechanism could underlie the reduced CD8 expression on CD8 + T cells in vivo during chronic HBV, HIV and SHIV infection and in response to mucosal HIV vaccination in mice [19] , [41] , [42] , [43] , [44] . The CD8 low cells described in these conditions show some functional similarities to the type 2-polarized CD8 low cells induced in vitro or in response to an IL-4-secreting tumour in vivo in the present study. The CpG methylation patterns observed here were remarkable in their spread and diversity. Changes in CpG methylation were seen across multiple regions of the Cd8a locus, and unique methylation signatures were identified in each T-cell population from DN3 cells onwards. These characteristics support a model in which differential methylation of multiple CpG sites contributes to the tuning of Cd8a transcription in response to different signals according to developmental stage (such as β-selection and positive selection in the thymus [45] ) and cytokines in the periphery [15] , [16] , [17] , [18] . At least five enhancers control CD8 expression during T-cell development and activation [46] , and numerous putative transcription factor binding sites are distributed throughout the Cd8a locus, including sites in and around the E8 V enhancer, promoter and gene body (K.L.H. and E.B.D., unpublished observations). Differential DNA methylation offers another potential layer of control to enable transmission of the CD8α expression profile to the next generation of cells. Of particular note, patterns of epigenetic modification and cytokine expression were flexible in some polarized effector T cells. Type 2 CD8 low cells could be induced to re-express CD8 and type 1 effector functions, and this reprogramming was accompanied by CpG demethylation at Cd8a , yielding a different pattern from either naive or typical IFN-γ-producing CD8 high cells. This epigenetic reprogramming of polarized effector CD8 + T cells occurred in cells that had already undergone many divisions in type 2 conditions and were able to maintain their CD8 low phenotype for an extended period in vivo . Clonal studies confirmed that the T cells which re-expressed CD8 were derived directly from CD8 low cells. Although commitment of CD4 + T cells to type 1 or type 2 cytokine expression commences within a few cell divisions after activation in polarizing conditions and is associated with epigenetic modification of multiple genes [47] , [48] , co-expression of cytokines of the alternative type has been induced in long-term polarized CD4 + T-cell populations in vivo [49] , [50] . We have also reported clonal lineage studies showing that some classical type 1 CD8 + T cells activated in vitro or in vivo retained the capacity to express type 2 cytokine genes in response to IL-4 (refs 51 , 52 ). Unlike these earlier studies in which CD4 + and CD8 + T cells acquired mixed type 1/2 profiles, in the present study most CD8 low cells lost type 2 functions when they re-expressed CD8 and acquired type 1 functions in response to IFN-γ. Thus, the extent to which type 1 and 2 lineage characteristics are merged might depend on the signals received, on the balance between the lineage-specifying transcription factors GATA-3 and T-bet [50] and on epigenetic signatures at these and effector genes [53] . In conclusion, we have identified remarkable epigenetic plasticity at the Cd8a locus, not only during T-cell ontogeny in the thymus but also in polarized effector CD8 + T cells, highlighting the capacity of the effector CD8 + T-cell response for heritable tuning of antigen sensitivity as well as effector function. Fluorescence-activated cell sorting and analysis Cells (no more than 2 × 10 7 cells per ml) were incubated on ice with fluorochrome-conjugated reagents: Ab to CD3ε (145-2C11, 1:400), CD8α (53-6.7, 1:600–1:1,000), CD8β (53-5.8, 1:400), CD4 (RM4-4, 1:1,000), CD24 (M1/69, 1:500), CD25 (7D4, 1:500), CD45.1 (A20, 1:200), CD49b (DX5, 1:200), TCRβ (H57-597, 1:200) and isotype controls (BD Pharmingen); Ab to B220 (RA3-6B2, 1:1,000), CD8α (53-6.7, 1:200–1:1,000), CD62L (MEL-14, 1:1,000), CD90.2 (53-2.1, 1:400), CD279 (PD-1; RMP1-30, 1:300), I-A b (AF6-120.1, 1:200), IFN-γ (XMG1.2, 1:200), IL-4 (11B11, 1:80-1:100) and isotype controls (BioLegend); Ab to CD4 (GK1.5, 1:1,000), CD11b (M1/70, 1:1,000), CD44 (IM7, 1:600), F4/80 (BM8, 1:500), Ter119 (TER-199, 1:900) and Vα2 (B20.1, 1:400) (eBioscience); Ab to human gzmB (GB12) and isotype control (Invitrogen); Ab to GATA-3 (TWAJ, 1:200) and isotype control with Foxp3 Staining Buffer Set (eBioscience). Cells were washed and purified using a FACSAria with FACSDiva software or analysed without sorting using a FACSCanto II with FACSDiva software (all BD Immunocytometry Systems). To minimize cell loss during processing, Ab staining of clonal populations was performed in 96-well V-bottom plates and supernatants were removed by pipette. In some instances, propidium iodide was added (100–200 ng ml −1 ; BD Pharmingen) for exclusion of dead cells. Post-acquisition data analyses were performed using FlowJo software (Tree Star). Cell isolation from mice Female C57BL/6 (CD45.2 + or congenic CD45.1 + ) mice (Animal Resources Centre, Murdoch, Australia) or B6.129(C)- Stat6 tm1Gru /J (STAT6 −/− ) mice (Professor Stephen Holdsworth, Monash Medical Centre, Clayton, Australia) were bred and housed under specific pathogen-free conditions at The University of Melbourne Department of Microbiology and Immunology (Parkville, Australia) and used at 6–8 weeks of age. Male OT-I (6 weeks of age) and RAG2 −/− γc −/− (8–10 weeks of age) mice were bred and housed at the QIMR Berghofer Medical Research Institute (Brisbane, Australia). All animal studies were approved by The University of Melbourne Animal Ethics Committee or the QIMR Berghofer Animal Ethics Committee as appropriate. Thymocytes were prepared by passing thymi through a 70-μm cell strainer. DP (CD4 + CD8 + ), CD4 SP (CD4 + CD8 − CD24 − ) and CD8 SP (CD4 − CD8 + CD24 − ) cells were purified by fluorescence-activated cell sorting. DN (CD4 − CD8 − ) thymocytes lacking lineage-specific markers (TCRβ − CD3ε − B220 − Ter119 − CD11b − CD49b − ) were separated into DN1 (CD25 − CD44 + ), DN2 (CD25 + CD44 + ), DN3 (CD25 + CD44 − ) and DN4 (CD25 − CD44 − ) subsets. Naive CD8 + T cells (CD8 + CD4 − CD44 low CD62L high ) and CD4 + T cells (CD4 + CD8 − CD44 low CD62L high ) were purified from pooled lymph nodes; the CD44 low population was defined as the 20% of cells with lowest CD44 expression. Generation and analysis of CD8 high and CD8 low T cells All cultures were performed in growth medium (RPMI 1640 with 1.8 mM L -glutamine, 0.88 mM sodium pyruvate, 88 mM MEM nonessential amino acids, 4.4 mM HEPES buffer, 88 U ml −1 penicillin, 88 U ml −1 streptomycin, 48 mM 2-mercaptoethanol and 7.9% heat-inactivated fetal calf serum). Where indicated, 5-azacytidine (Sigma) in DMSO, or DMSO alone, was added. For primary activation in T75 flasks, naive CD8 + T cells were cultured in 30 ml at 1 × 10 5 (for analysis at day 4), 4.5 × 10 4 (day 7) or 2 × 10 4 (day 10) cells per flask coated with Ab to CD3ε (10 μg ml −1 ; 145-2C11), CD8α (10 μg ml −1 ; 53.6) and CD11a (5 μg ml −1 ; I21/7.7). For primary activation in 24-well plates, plates were coated with Ab as above, and cells were cultured in 2 ml at 2 × 10 5 (for analysis at day 2), 2 × 10 4 (day 4), 1 × 10 3 (day 5), 1 × 10 4 (day 6) or 5 × 10 3 (day 8, 10) cells per well. Cultures were performed in growth medium with human recombinant IL-2 (10 U ml −1 ; Roche Diagnostics) (neutral conditions) or IL-2, mouse recombinant IL-4 (25 ng ml −1 ; ProSpec-Tany TechnoGene) and anti-IFN-γ Ab (1 μg ml −1 ; XMG1.2) (type 2 polarizing conditions). In some experiments, IL-13 (ProSpec-Tany TechnoGene) was added. For secondary stimulation, activated CD8 high or CD8 low cells were purified by Ficoll-Paque separation and sorting once (>98% purity) or twice (≥99.9% purity) for high or low CD8α expression, with exclusion of dead cells based on forward scatter and propidium iodide uptake. Cells were cultured at 4.48 × 10 4 (day 6 analyses) or 2.24 × 10 4 (day 10) cells per well in 6 ml in six-well plates, or at 1 × 10 5 (day 2), 5 × 10 4 (day 4), 1 × 10 4 (day 6) or 5 × 10 3 (days 8, 10 and 12) cells per well in 2 ml in 24-well plates. Wells were coated with anti-CD3ε/CD8/CD11a Ab as above, except that anti-CD3ε Ab was reduced to 1 μg ml −1 , in neutral or type 2 conditions, or with IL-2 and anti-mouse IL-4 Ab (10 μg ml −1 ; 11B11) or IFN-γ (2 ng ml −1 ; ProSpec-Tany TechnoGene) or both (reversal conditions). For cloning, individual cells were sorted twice and on the second sort deposited directly into 96-well round-bottomed plates with the indicated stimuli in 200 μl growth medium. Effector phenotype was determined by re-culturing cells from 7-day primary or 10-day secondary cultures with IL-2 alone for 2 or 3 days, respectively, then adding phorbol 12-myristate 13-acetate (PMA; 10 ng ml −1 ), ionomycin (500 ng ml −1 ) (both Sigma) and GolgiStop (0.67 μl ml −1 ; BD Biosciences) for 4 h. Cells were purified by Ficoll-Paque separation, stained for surface CD8α, fixed and permeabilized using Cytofix/cytoperm kit reagents (BD Biosciences), then stained for intracellular IFN-γ, IL-4 and granzyme B. Adoptive transfer of CD8 high and CD8 low cells Naive CD45.1 + CD8 + T cells were activated in anti-CD3ε/CD8/CD11a Ab-coated flasks (3 × 10 4 cells per flask) under neutral or type 2 conditions for 7 days, then rested in IL-2 alone for 2 days. Ficoll-Paque-separated CD8 high cells from neutral cultures or CD8 low cells from type 2 cultures were purified and transferred into CD45.2 + mice (2.5 × 10 6 cells per mouse intraperitoneally, 3 mice per group). After 62 days, cell suspensions were prepared from pooled spleen and lymph nodes of individual recipient mice. Donor CD45.1 + cells were labelled with anti-CD45.1-PE Ab in the presence of 2.4G2 hydridoma supernatant (containing mAb against murine Fcγ receptors II and III with 0.5% normal mouse serum and 0.5% normal rat serum) and enriched from suspensions using MACS anti-PE microbeads (Miltenyi Biotech). CD8 high or CD8 low CD45.1 + cells (B220 − CD4 − F4/80 − I-A b− CD90.2 + CD44 high phenotype) were enumerated and purified by flow cytometry. Cells isolated from individual mice were pooled for extraction of genomic DNA. In vivo activation of CD8 + T cells CD8 + T cells were purified from OT-I (243.2) mice using MACS CD8 microbeads (Miltenyi Biotech) (97% CD8 + Vα2 + after purification); 2.4 × 10 6 were coinjected into RAG2 −/− γc −/− mice with 3.5 × 10 7 OVA-expressing tumour cells expressing IL-4 (EG7-IL-4 + ) or control vector (EG7-IL-4 − ) [18] in 200 μl saline subcutaneously at the base of the tail. EG7-IL-4 + tumour recipients also received 250 μg purified anti-IFN-γ mAb (XMG1.2) intraperitoneally on days 0, 4 and 6. Splenocytes were isolated 9 days later for purification and analysis. DNA extraction and analysis of CpG methylation Genomic DNA was extracted from 1.6 × 10 4 –2 × 10 5 cells using a QIAamp DNA kit (Qiagen), with additional wash steps to remove protein contaminants. Bisulphite conversion was performed on 90–500 ng sheared genomic DNA using a MethylCode Bisulfite Conversion Kit (Invitrogen); the DNA was then used as template in one or two rounds of nested PCR using primers to amplify eight regions of the bisulphite-modified Cd8a locus. PCR amplification of bisulphite-treated DNA was performed in 50 μl reactions in an Eppendorf MasterCycler Pro S with GoTaq (Promega), 20 pmole sense and anti-sense primers (Invitrogen), HPLC water (Burdick and Jackson) and either 3–5 μl of bisulphite-modified DNA (first-round PCR) or 3–5 μl of the first-round PCR reaction (second-round PCR). Primers and touchdown PCR conditions optimized for each primer pair are shown in Supplementary Table 2 . Final-round PCR products were gel-purified using a QIAquick gel extraction kit (Qiagen) and individual products were cloned in DH5α bacterial cells using a pGEMT-easy vector system (Promega). Cloned products were amplified from individual bacterial colonies by PCR (25 μl reaction in 96-well PCR plates (Eppendorf)) with GoTaq, 20 pmole sense and anti-sense vector primers (5′: 5′-gtaaaacgacggccag-3′; 3′: 5′-caggaaacagctatgac-3′) and HPLC water. PCR conditions were 95 °C for 5 min, 33 cycles of 95 °C for 30 s, 57 °C for 30 s and 72 °C for 1 min, followed by 95 °C for 1 min, 57 °C for 1 min and 72 °C for 7 min. Amplified products were treated with ExoSAP-IT reagent (USB Corporation) and subsequently used in 20 μl sequencing reactions with Big Dye v3.1, Big Dye v3.1 sequencing buffer (both Applied Biosystems), 5% DMSO, 20 pmole anti-sense vector primer and HPLC water. Sequencing PCR conditions were 95 °C for 5 min, followed by 30 cycles of 96 °C for 10 s, 50 °C for 10 s and 60 °C for 4 min. Products were purified using a Dye Ex 96-well kit (Qiagen) or NucleoSEQ Columns (Macherey-Nagel), dried at 90–95 °C for ~30 min and submitted to Molecular Diagnostics (Centre for Translational Pathology, The University of Melbourne) for sequence determination. Sequences from clones were analysed using CLC Sequence Viewer 6 (CLC bio A/S) and FinchTV (Geospiza) to verify the methylation status of CpG cytosines. At least 10 complete sequences were obtained for each region of Cd8a for each population analysed. Statistical analyses Data were analysed using GraphPad Prism, Microsoft Excel and IBM SPSS software. Where required, a Kolmogorov–Smirnov test with the Dallal–Wilkinson–Lillie for corrected P -value was used to determine whether populations were normally distributed. How to cite this article: Harland, K. L. et al. Epigenetic plasticity of Cd8a locus during CD8 + T-cell development and effector differentiation and reprogramming. Nat. Commun. 5:3547 doi: 10.1038/ncomms4547 (2014).